Fibroblast growth factor 21 protects against cardiac hypertrophy in mice Fibroblast growth factor 21 is an endocrine factor, secreted mainly by the liver, that exerts metabolic actions that favour glucose metabolism. Its role in the heart is unknown. Here we show that Fgf21 −/− mice exhibit an increased relative heart weight and develop enhanced signs of dilatation and cardiac dysfunction in response to isoproterenol infusion, indicating eccentric hypertrophy development. In addition, Fgf21 −/− mice exhibit enhanced induction of cardiac hypertrophy markers and pro-inflammatory pathways and show greater repression of fatty acid oxidation. Most of these alterations are already present in Fgf21 −/− neonates, and treatment with fibroblast growth factor 21 reverses them in vivo and in cultured cardiomyocytes. Moreover, fibroblast growth factor 21 is expressed in the heart and is released by cardiomyocytes. Fibroblast growth factor 21 released by cardiomyocytes protects cardiac cells against hypertrophic insults. Therefore, the heart appears to be a target of systemic, and possibly locally generated, fibroblast growth factor 21, which exerts a protective action against cardiac hypertrophy. Cardiac hypertrophy and subsequent progression to heart failure represents a major cause of morbidity and mortality. The defining features of cardiac hypertrophy are an increase in cardiomyocyte (CM) size, enhanced protein synthesis, a greater degree of sarcomere organization and a shift from fatty acids to glucose as an energy source [1] . Chronic inflammation has an important role in hypertrophic responses in the heart [2] , [3] . Heart failure remains a critical health problem and the identification of underlying molecular targets and novel protective agents is of crucial importance for improving preventive and therapeutic strategies. Communication among cardiac cells via secreted factors may contribute to myocardial hypertrophic remodelling [4] , [5] . The term cardiomyokine has emerged to describe proteins secreted from the heart that have autocrine, paracrine and/or endocrine functions crucial for the maintenance of cardiac function [6] . The number of cardiomyokines has been estimated at between 30 and 60 (refs 7 , 8 ). Because of their extracellular localization, secreted cardiomyokines, show promise as therapeutic targets, or possibly even therapeutic agents. Fibroblast growth factor 21 (FGF21), a secreted protein that acts as a metabolic regulator, is involved in the control of glucose homeostasis, insulin sensitivity and ketogenesis [9] , [10] . The liver is considered the main site of production and release of FGF21 into the blood [9] , [11] , but extra-hepatic tissues, such as white adipose tissue (WAT) and brown adipose tissue (BAT) and skeletal muscle also express FGF21 (refs 12 , 13 , 14 ). The endocrine actions of FGF21 are involved in the activation of BAT thermogenesis [15] and the promotion of glucose uptake by white adipocytes [16] . FGF21 also has autocrine/paracrine effects, inducing hepatic ketogenesis [9] and promoting sensitization to antidiabetic agents in WAT [17] . The cellular actions of FGF21 are mediated by FGF receptors (mainly FGFR1 and FGFR4 in adipose tissues and liver, respectively) and β-Klotho, a single-pass transmembrane protein that functions as an obligate coreceptor for FGF21 signalling [18] , [19] . Despite the importance of FGF21 as an endocrine factor, to date, no studies have focused directly on the role of FGF21 in the heart. In the present study, we analyse the role of FGF21 in cardiac tissue. We observe that mice lacking FGF21 are more prone to develop cardiac hypertrophy, and treatment of these mice with FGF21 protects against hypertrophic responses. Moreover, the signals that promote hypertrophy induce cardiac FGF21 expression and protein secretion in vivo and in vitro . Cardiac hypertrophy is enhanced in Fgf21 −/− mice We first undertook an analysis of the role of FGF21 in the heart by determining the impact of FGF21 ablation ( Fgf21 −/− ) in mice. Fgf21 −/− mice did not show marked alterations in morphometric, metabolic or endocrine profiles under basal, fed conditions, in agreement with previous reports of independently generated mouse models of FGF21 gene invalidation ( Supplementary Tables S1 and S2 ). We compared the morphology of hearts from adult Fgf21 −/− mice at baseline and after 7 days of exposure to continuous isoproterenol infusion to induce cardiac hypertrophy. 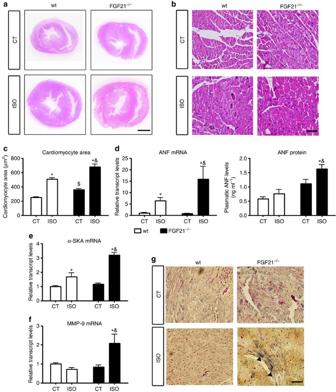Figure 1: Cardiac hypertrophy is enhanced inFgf21-null mice. Adult wild-type (wt; white bars) andFGF21−/−mice (black bars) were continuously infused with isoproterenol (ISO) for 7 days to experimentally induce heart hypertrophy. (a) Representative two-cardiac chamber (axial) histological sections of hearts stained with H&E. Scale bar, 1 mm. (b) Magnified ( × 20) images of histological sections in (a) used to determine CM cross-sectional area (CSA). Scale bar, 50 μm. (c) Quantification of CM cross-sectional area in the left ventricular wall. (d) mRNA expression and plasma protein levels of the hypertrophy marker ANF. mRNA expression levels of the hypertrophy marker α-SKA (e) and fibrosis marker matrix metalloproteinase-9 (MMP-9) (f). (g) Determination of fibrosis in histological sections by Masson’s Trichrome staining. Original magnification, × 20. Scale bar, 50 μm. Arrows show fibrotic areas (blue). Results are expressed as means±s.e.m.,n=4–5 mice per group. Data were analysed by one-way ANOVA (*P<0.05 compared with corresponding control [CT] mice;$P<0.05 compared with wild-type CT mice;&P<0.05 compared with wild-type isoproterenol-treated mice). In control animals, total heart weight (HW), as well as HW expressed relative to body weight (HW/BW) and tibia length (HW/TL) were significantly higher in Fgf21 −/− mice than in wild-type mice ( Table 1 ). After 7 days of isoproterenol infusion, HW was significantly increased in both wild-type and Fgf21 −/− mice. The increase in HW was more pronounced in isoproterenol-treated Fgf21 −/− mice than in isoproterenol-treated wild-type mice, whether expressed as HW/TL or HW/BW. No differences in blood pressure or heart rate were found under any conditions tested ( Supplementary Table S3 ). Under basal conditions, diastolic and systolic interventricular septum and posterior wall thickness, determined by echocardiography ( Table 1 and Supplementary Table S4 ), were not significantly different between wild-type and Fgf21 −/− mice. Isoproterenol significantly increased interventricular septum thickness and posterior wall thickness in Fgf21 −/− mice during diastole. Histological examination of hematoxylin and eosin (H&E)-stained left ventricle (LV) tissue sections revealed that the CM cross-sectional area was larger in Fgf21 −/− than in wild-type mice ( Fig. 1a–c and Supplementary Table S5 ). Isoproterenol treatment significantly increased cross-sectional area in both Fgf21 −/− and wild-type mice but the increase in cross-sectional area after isoproterenol was greater in Fgf21 −/− mice. Table 1 Morphometric and echocardiography data from wild-type and FGF21 −/− mice after ISO-induced hypertrophy. Full size table Figure 1: Cardiac hypertrophy is enhanced in Fgf21 -null mice. Adult wild-type (wt; white bars) and FGF21 −/− mice (black bars) were continuously infused with isoproterenol (ISO) for 7 days to experimentally induce heart hypertrophy. ( a ) Representative two-cardiac chamber (axial) histological sections of hearts stained with H&E. Scale bar, 1 mm. ( b ) Magnified ( × 20) images of histological sections in ( a ) used to determine CM cross-sectional area (CSA). Scale bar, 50 μm. ( c ) Quantification of CM cross-sectional area in the left ventricular wall. ( d ) mRNA expression and plasma protein levels of the hypertrophy marker ANF. mRNA expression levels of the hypertrophy marker α-SKA ( e ) and fibrosis marker matrix metalloproteinase-9 (MMP-9) ( f ). ( g ) Determination of fibrosis in histological sections by Masson’s Trichrome staining. Original magnification, × 20. Scale bar, 50 μm. Arrows show fibrotic areas (blue). Results are expressed as means±s.e.m., n =4–5 mice per group. Data were analysed by one-way ANOVA (* P <0.05 compared with corresponding control [CT] mice; $ P <0.05 compared with wild-type CT mice; & P <0.05 compared with wild-type isoproterenol-treated mice). Full size image In wild-type mice, isoproterenol increased systolic LV internal diameter and end-systolic volume ( Table 1 ). In Fgf21 −/− mice, isoproterenol infusion led to a significant increase in both end-diastolic and end-systolic LV internal diameter and volumes (end-diastolic volume and end-systolic volume), an increase significantly higher than in wild-type mice. The H/R ratio, a measure of concentric versus eccentric cardiac hypertrophy, was decreased in the Fgf21 −/− mice after isoproterenol infusion, indicating eccentric cardiac hypertrophic response. The sphericity index was also decreased in the Fgf21 −/− mice in response to isoproterenol. Finally, LV ejection fraction and fractional shortening were not affected by isoproterenol in wild-type mice, but both parameters were significantly decreased by isoproterenol treatment in Fgf21 −/− mice. The expression of the hypertrophic markers atrial natriuretic factor (ANF) and α-skeletal actin (α-SKA) mRNAs, was similar in wild-type and Fgf21 −/− mice under basal conditions ( Fig. 1d ). Isoproterenol infusion caused an increase in ANF mRNA and plasma protein and α-SKA mRNA, an effect that was significantly more pronounced in Fgf21 −/− mice than in wild-type mice. To assess fibrosis, we performed Masson’s Trichrome staining and evaluated the expression of matrix metalloproteinase-9 ( Fig. 1f ). By both measures, isoproterenol led to a substantial increase in fibrosis in Fgf21 −/− mice but not in wild-type mice. Collectively, it is concluded that the lack of FGF21 promotes cardiac hypertrophy and sensitizes mice to hypertrophic stimuli and associated derangements such as fibrosis. Cardiac inflammatory signals and metabolism in Fgf21 −/− mice Considering that a pro-inflammatory status is often associated with cardiac hypertrophy development, we investigated the effects of the absence of FGF21 on cardiac expression of pro-inflammatory marker genes, nuclear factor-kappaB (NF-κB) activity, and pro-inflammatory plasma cytokine levels in response to isoproterenol. We measured transcript levels for the cytokines interleukin-6 (IL-6), tumour necrosis factor-α (TNFα) and monocyte chemoattractant protein-1 (MCP-1) ( Fig. 2a ). With the exception of TNFα, inflammatory gene expression was significantly higher in Fgf21 −/− mice than in wild-type mice before treatment. The expression of inflammatory genes was markedly increased in both wild-type and Fgf21 −/− mice in association with isoproterenol treatment-induced cardiac hypertrophy; however, under these conditions, IL-6 and MCP-1 mRNA levels were significantly higher in Fgf21 −/− mice than in wild-type mice. A similar pattern was observed for plasma levels of IL-6 and MCP-1 ( Fig. 2b ). Moreover, NF-κB activity in the hearts of Fgf21 −/− mice was elevated under basal conditions and following isoproterenol infusion ( Fig. 2c ). 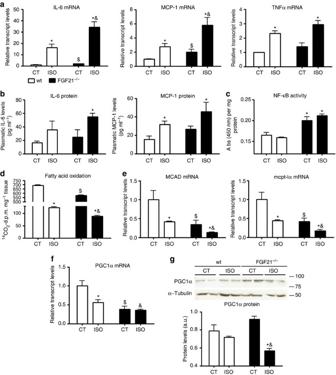Figure 2: Cardiac inflammatory signals and metabolism inFgf21−/−mice. (a) mRNA expression levels of the pro-inflammatory genesIL-6,MCP-1andTNFα. (b) Plasma protein levels of IL-6 and MCP-1. (c) NF-κB activity in nuclear extracts from hearts. (d) FAO rates in homogenates from freshly isolated hearts. (e) mRNA expression levels of the lipid catabolism genesMCADandmcpt-Iα. (f) mRNA level of PGC1α. (g) PGC1α protein levels in nuclear extracts from hearts. Top: representative images from western-blots; bottom: protein quantification. Results are expressed as means±s.e.m.,n=4–5 mice per group. Data were analysed by one-way ANOVA (*P<0.05 compared with corresponding control [CT] mice;$P<0.05 compared with wild-type (wt) CT mice;&P<0.05 compared with wild-type isoproterenol-treated mice). Figure 2: Cardiac inflammatory signals and metabolism in Fgf21 −/− mice. ( a ) mRNA expression levels of the pro-inflammatory genes IL-6 , MCP-1 and TNFα . ( b ) Plasma protein levels of IL-6 and MCP-1. ( c ) NF-κB activity in nuclear extracts from hearts. ( d ) FAO rates in homogenates from freshly isolated hearts. ( e ) mRNA expression levels of the lipid catabolism genes MCAD and mcpt-Iα . ( f ) mRNA level of PGC1α. ( g ) PGC1α protein levels in nuclear extracts from hearts. Top: representative images from western-blots; bottom: protein quantification. Results are expressed as means±s.e.m., n =4–5 mice per group. Data were analysed by one-way ANOVA (* P <0.05 compared with corresponding control [CT] mice; $ P <0.05 compared with wild-type (wt) CT mice; & P <0.05 compared with wild-type isoproterenol-treated mice). Full size image Considering the close association between impaired fatty acid oxidation (FAO) and cardiac hypertrophy, we examined FAO rates as well as the expression of FAO-associated genes and PPARγ coactivator-1α (PGC1α). The FAO rate was significantly reduced in Fgf21 −/− mice compared with wild-type mice under both basal and isoproterenol-infusion conditions ( Fig. 2d ). Moreover, transcript levels of the FAO-related genes carnitine palmitoyltransferase ( mcpt)-Iα and medium-chain acyl-CoA dehydrogenase ( MCAD ), as well as those of PGC1α were markedly decreased in Fgf21 −/− mice under basal conditions; after isoproterenol, expression levels were downregulated in both wild-type and Fgf21 −/− mice ( Fig. 2e ). However, the levels of PGC1α, MCAD and mcpt-Iα mRNA in isoproterenol-infused mice were significantly lower in Fgf21 −/− mice than in wild-type mice. The levels of PGC1α protein were also lower in Fgf21 −/− mice than in wild-type mice infused with isoproterenol ( Fig. 2g ). Overall these findings indicate that the absence of FGF21 and subsequent cardiac hypertrophy are associated with enhanced pro-inflammatory signalling and repression of FAO pathways. FGF21 protects against cardiac hypertrophy in vivo In order to ascertain whether enhanced cardiac hypertrophy in Fgf21 −/− mice was a pathological consequence of progressive processes acting throughout the life of the mouse or was a more primary event that occurred before putative long-acting metabolic challenges, we analysed hearts from Fgf21 −/− mice in the immediate neonatal period ( Fig. 3a ). Although absolute values for BW and HW were not different between the two genotypes owing to individual variability within each experimental group, the HW/BW ratio for individuals did change (See supplementary Table S6 ). The increase in HW/BW ratio (ΔHW/BW) in response to isoproterenol was significantly enhanced in Fgf21 −/− mice compared with wild-type mice, indicating that, in the absence of FGF21, the hypertrophic response to isoproterenol in the heart is enhanced ( Fig. 3b ). Administration of FGF21 prevented the increase in HW/BW in wild-type and Fgf21 −/− mice. Consistent with heart enlargement, the CM cross-sectional area in the LV wall was also increased in isoproterenol-treated mice, and the increase was significantly higher in Fgf21 −/− neonates than in wild-type pups. FGF21 significantly reduced isoproterenol-induced CM enlargement in wild-type and Fgf21 −/− mice ( Fig. 3c ). 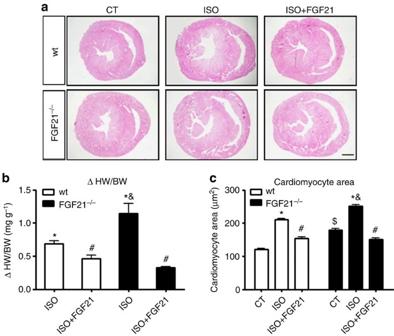Figure 3: FGF21 prevents the development of cardiac hypertrophyin vivo. Six-day-old wild-type (wt; white bars) andFGF21−/−mice (black bars) were injected (i.p.) with isoproterenol (ISO) for 7 days (alone or combination with FGF21) to induce cardiac hypertrophy. (a) Representative two-cardiac chamber (axial) histological sections of hearts stained with H&E. Scale bar, 600 μm. (b) HW/BW, expressed in milligrams per gram. (c) Quantification of the CM cross-sectional area (CSA) in the left ventricular wall. Results are expressed as means±s.e.m.,n=3–6 mice per group. Data were analysed by one-way ANOVA (*P<0.05 compared with corresponding control [CT] mice;#P<0.05 compared with corresponding isoproterenol-treated mice;$P<0.05 compared with wild-type CT mice;&P<0.05 compared with wild-type isoproterenol-treated mice). Figure 3: FGF21 prevents the development of cardiac hypertrophy in vivo . Six-day-old wild-type (wt; white bars) and FGF21 −/− mice (black bars) were injected (i.p.) with isoproterenol (ISO) for 7 days (alone or combination with FGF21) to induce cardiac hypertrophy. ( a ) Representative two-cardiac chamber (axial) histological sections of hearts stained with H&E. Scale bar, 600 μm. ( b ) HW/BW, expressed in milligrams per gram. ( c ) Quantification of the CM cross-sectional area (CSA) in the left ventricular wall. Results are expressed as means±s.e.m., n =3–6 mice per group. Data were analysed by one-way ANOVA (* P <0.05 compared with corresponding control [CT] mice; # P <0.05 compared with corresponding isoproterenol-treated mice; $ P <0.05 compared with wild-type CT mice; & P <0.05 compared with wild-type isoproterenol-treated mice). Full size image Expression of ANF and α-SKA were also induced in isoproterenol-treated neonates ( Fig. 4a ), and the induction of ANF expression was significantly more pronounced in Fgf21 −/− pups. FGF21 significantly attenuated isoproterenol-induced α-SKA expression in wild-type mice and decreased expression of both ANF and α-SKA in Fgf21 −/− neonates. In addition, IL-6 mRNA levels were significantly increased in hearts from isoproterenol-treated neonates, but were more markedly elevated in Fgf21 −/− pups. FGF21 treatment significantly attenuated the expression of IL-6 in Fgf21 −/− mice. A similar pattern was found in the plasma levels of ANF and IL-6 ( Fig. 4b ). Finally, the FAO-associated genes mcpt-Iα and MCAD were upregulated after FGF21 treatment in Fgf21 −/− mice ( Fig. 4c ). PGC1α mRNA levels were downregulated after isoproterenol-induced cardiac hypertrophy only in Fgf21 −/− mice and were restored after FGF21 treatment. 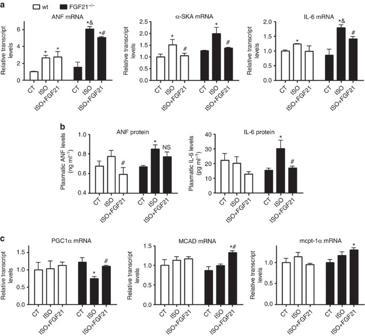Figure 4: Cardiac gene expression and plasma levels inFgf21−/−neonates. (a) mRNA expression levels of the hypertrophy markers ANF and α-SKA and pro-inflammatory marker IL-6. (b) Plasma protein levels of ANF and IL-6. (c) mRNA expression levels of PGC1α and lipid catabolism genesMCADandmcpt-Iα. Results are expressed as means±s.e.m.,n=3–6 mice per group. Data were analysed by one-way ANOVA (*P<0.05 compared with corresponding control [CT] mice;#P<0.05 compared with corresponding isoproterenol-treated mice;$P<0.05 compared with wild-type (wt) CT mice;&P<0.05 compared with wild-type isoproterenol-treated mice). NS, not significant. Figure 4: Cardiac gene expression and plasma levels in Fgf21 −/− neonates. ( a ) mRNA expression levels of the hypertrophy markers ANF and α-SKA and pro-inflammatory marker IL-6. ( b ) Plasma protein levels of ANF and IL-6. ( c ) mRNA expression levels of PGC1α and lipid catabolism genes MCAD and mcpt-Iα . Results are expressed as means±s.e.m., n =3–6 mice per group. Data were analysed by one-way ANOVA (* P <0.05 compared with corresponding control [CT] mice; # P <0.05 compared with corresponding isoproterenol-treated mice; $ P <0.05 compared with wild-type (wt) CT mice; & P <0.05 compared with wild-type isoproterenol-treated mice). NS, not significant. Full size image FGF21 directly targets cardiac cells In order to establish whether the effects of FGF21 observed in in vivo studies involved a direct action of FGF21 on cardiac cells, we used cultured rat neonatal CMs (NCMs). Phenylephrine treatment increased cross-sectional area, an indication of hypertrophy, and FGF21 significantly attenuated the phenylephrine-induced cell enlargement ( Fig. 5a ). Transcript levels of ANF and α-SKA were increased in association with phenylephrine, and this effect was reduced by treatment with FGF21 ( Fig. 5b ). Exposure of NCMs to phenylephrine significantly decreased PGC1α mRNA levels and induced an increase in IL-6 mRNA levels; both effects were abrogated by FGF21 treatment. Moreover, exposure of NCMs to FGF21 attenuated the formation of reactive oxygen species (ROS) and stimulation of NF-κB activity induced by phenylephrine ( Fig. 5c ). 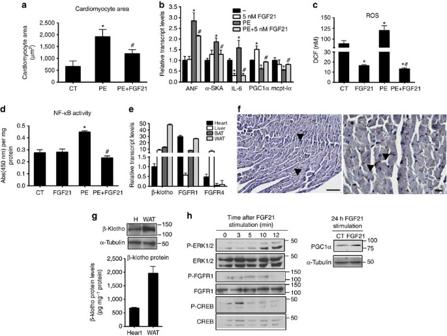Figure 5: FGF21 protects CMs against phenylephrine-induced hypertrophy. (a) CM cross-sectional area (CSA) and (b) mRNA expression levels in neonatal CMs (NCMs) after phenylephrine (PE)-induced hypertrophy alone or with FGF21 pretreatment (5 nM) for 24 h. (c) ROS levels and (d) NF-κB activity in NCMs. (e) mRNA levels of FGF receptors (FGFR1, FGFR4) and coreceptor β-Klotho. (f) Detection of β-Klotho in paraffin sections of the heart by immunohistochemistry. Left: original magnification, × 20. Scale bar, 100 μm. Right: original magnification × 50. Scale bar, 50 μm. Arrows indicate β-Klotho staining (brown). (g) β-Klotho protein levels (pg mg−1protein) quantified by ELISA, and a representative immunoblot showing the levels of β-Klotho protein in the heart and in WAT. (h) Representative western blot of P-ERK1/2, ERK1/2, P-FGFR1, FGFR1, P-CREB, CREB and PGC1α in NCMs stimulated with 5 nM FGF21 at different time points. Data are presented as means±s.e.m. Each experiment was conducted in triplicate in at least two independent CM isolations. Data were analysed by one-way ANOVA (*P<0.05 compared with control cells;#P<0.05 compared with phenylephrine-treated cells). Figure 5: FGF21 protects CMs against phenylephrine-induced hypertrophy. ( a ) CM cross-sectional area (CSA) and ( b ) mRNA expression levels in neonatal CMs (NCMs) after phenylephrine (PE)-induced hypertrophy alone or with FGF21 pretreatment (5 nM) for 24 h. ( c ) ROS levels and ( d ) NF-κB activity in NCMs. ( e ) mRNA levels of FGF receptors (FGFR1, FGFR4) and coreceptor β-Klotho. ( f ) Detection of β-Klotho in paraffin sections of the heart by immunohistochemistry. Left: original magnification, × 20. Scale bar, 100 μm. Right: original magnification × 50. Scale bar, 50 μm. Arrows indicate β-Klotho staining (brown). ( g ) β-Klotho protein levels (pg mg −1 protein) quantified by ELISA, and a representative immunoblot showing the levels of β-Klotho protein in the heart and in WAT. ( h ) Representative western blot of P-ERK1/2, ERK1/2, P-FGFR1, FGFR1, P-CREB, CREB and PGC1α in NCMs stimulated with 5 nM FGF21 at different time points. Data are presented as means±s.e.m. Each experiment was conducted in triplicate in at least two independent CM isolations. Data were analysed by one-way ANOVA (* P <0.05 compared with control cells; # P <0.05 compared with phenylephrine-treated cells). Full size image To further investigate the effects of FGF21 in the inflammatory process, we studied the influence of FGF21 on the cardiac response to lipopolysaccharide (LPS) ( Supplementary Fig. S1 ). FGF21 significantly reduced LPS-induced expression of pro-inflammatory genes in NCMs. Results obtained in vivo indicated that cardiac transcript levels and plasma protein levels of IL-6 and MCP-1 were significantly enhanced in Fgf21 −/− mice compared with wild-type mice following LPS injection. Overall, a protective role of FGF21 against the induction of inflammation was confirmed. Given the evidence of direct effects of FGF21 on cardiac cells, we further analysed the expression levels of FGF21 receptors (FGFR1 and -R4) and coreceptor (β-Klotho) in the heart compared with that in liver, BAT and WAT. We detected transcripts for both FGFR1 and -R4 and the coreceptor β-Klotho in the heart ( Fig. 5e ). The most highly expressed FGF receptor form was FGFR1, which was found at levels at least as high as those in adipose tissues, whereas FGFR4 was less abundant, in agreement with previous reports [20] . Transcript levels of β-Klotho, which is considered to confer specific responsiveness to FGF21, were less abundant in the heart than in other tissues analysed ( Fig. 5e ). However, immunohistochemistry confirmed the presence of β-Klotho in the heart ( Fig. 5f ). Western blot analysis also showed that β-Klotho protein was expressed at lower levels in the heart than in other FGF21 target tissues such as WAT ( Fig. 5g ), although the difference was less marked at the protein level than at the mRNA level. Using specific ELISAs to quantify these differences, we found β-Klotho levels in the heart were about one-third those in WAT. Finally, in order to further confirm that FGF21 acts directly on cardiac cells, we analysed the activation of FGFR1 and the MAP kinase cascade, bona fide indicators of a β-Klotho/FGF receptor-dependent cellular response to FGF21 (ref. 21 ). The results indicated that FGF21 induced the phosphorylation of FGFR1 and ERK (extracellular signal-regulated kinase)-1/2 in NCMs ( Fig. 5h ), confirming that cardiac cells are genuine targets of FGF21. Moreover, we found that FGF21 treatment also induced CREB phosphorylation and increased PGC1α protein levels. FGF21 is expressed and secreted by cardiac cells Considering that, to date, FGF21 target tissues are, in turn, FGF21-producing tissues, we sought to determine whether the heart is also an FGF21-producing tissue. The adult heart expressed the FGF21 transcript, although at lower levels compared with other tissues such as liver and WAT ( Supplementary Fig. S2A ). FGF21 mRNA expression in the heart was rapidly induced during the transition from the fetal to neonatal period; in fact, FGF21 expression levels in hearts from 1-day-old pups were similar to those in adult hearts ( Fig. 6a ). Treatment with isoproterenol significantly increased the expression levels of FGF21 mRNA in the heart ( Fig. 6b and Supplementary Fig. S2B ). Other pathological cardiac interventions, such as transverse aortic constriction (TAC) and myocardial infarction (MI), induced mRNA expression in the heart, whereas ischaemia/reperfusion (I/R) did not, probably due to the short-term nature of this intervention (1 day) ( Fig. 6b ). Isolation of cardiac cells from adult hearts confirmed that FGF21 was mainly expressed by the CM fraction ( Fig. 6c ), rather than in non-cardiac (non-CM) cells in which the FGF21 transcript was almost undetectable. The expression levels of FGF21 in cardiac fibroblasts were also much lower than in CMs. 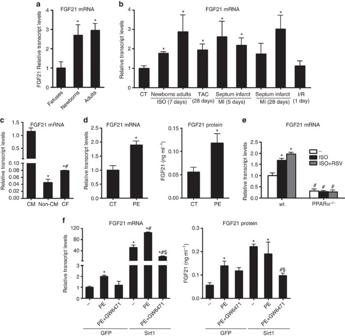Figure 6: FGF21 is expressed and released by cardiac cells. (a) FGF21 expression levels in fetuses (18 days), newborns (1 day old) and adult mice (4 months old);n=5 mice per group. (b) FGF21 mRNA levels in the heart after different interventions to induce cardiac damage: cardiac hypertrophy induced by isoproterenol (ISO) (7days) and TAC (28 days); early (5 days) and late (28 days) MI in the septum or in the left ventricle infarcted area; and 1 day reperfusion after 30 min ischemia;n=5 mice per group. (c) FGF21 mRNA levels in the CM, non-CM (Non-CM) and cardiac fibroblast (CF) fractions from isolated adult wild-type (wt) mouse hearts. (d) FGF21 mRNA levels in neonatal CMs (NCMs) and protein levels in culture media after phenylephrine (PE) stimulation for 24 h. (e) FGF21 mRNA levels in wild-type andPPARα−/−mice injected with isoproterenol (i.p.) for 7 days;n=5 mice per group. (f) NCMs overexpressing Sirt1 or GFP control vector (10 IFU per cell) were treated with phenylephrine and the PPARα antagonist GW6471 (1 μM), alone or in combination, for 24 h. Results are expressed as means±s.e.m.. Thein vitroexperiments were conducted in triplicate in at least two independent CM isolations. Data were analysed by one-way ANOVA (*P<0.05 compared with wild-type (wt) control mice, cells or CM fraction [C];#P<0.05 compared with isoproterenol-treated wild-type animals [E], Ad-Sirt1-infected control cells [F] or Non-CM [C];$P<0.05 compared with Ad-Sirt1-infected phenylephrine-stimulated cells [F]). Figure 6: FGF21 is expressed and released by cardiac cells. ( a ) FGF21 expression levels in fetuses (18 days), newborns (1 day old) and adult mice (4 months old); n =5 mice per group. ( b ) FGF21 mRNA levels in the heart after different interventions to induce cardiac damage: cardiac hypertrophy induced by isoproterenol (ISO) (7days) and TAC (28 days); early (5 days) and late (28 days) MI in the septum or in the left ventricle infarcted area; and 1 day reperfusion after 30 min ischemia; n =5 mice per group. ( c ) FGF21 mRNA levels in the CM, non-CM (Non-CM) and cardiac fibroblast (CF) fractions from isolated adult wild-type (wt) mouse hearts. ( d ) FGF21 mRNA levels in neonatal CMs (NCMs) and protein levels in culture media after phenylephrine (PE) stimulation for 24 h. ( e ) FGF21 mRNA levels in wild-type and PPARα −/− mice injected with isoproterenol (i.p.) for 7 days; n =5 mice per group. ( f ) NCMs overexpressing Sirt1 or GFP control vector (10 IFU per cell) were treated with phenylephrine and the PPARα antagonist GW6471 (1 μM), alone or in combination, for 24 h. Results are expressed as means±s.e.m.. The in vitro experiments were conducted in triplicate in at least two independent CM isolations. Data were analysed by one-way ANOVA (* P <0.05 compared with wild-type (wt) control mice, cells or CM fraction [C]; # P <0.05 compared with isoproterenol-treated wild-type animals [E], Ad-Sirt1-infected control cells [F] or Non-CM [C]; $ P <0.05 compared with Ad-Sirt1-infected phenylephrine-stimulated cells [F]). Full size image Our analysis of FGF21 expression in NCMs showed that FGF21 mRNA levels were significantly increased following exposure to phenylephrine ( Fig. 6d ). Finally, to determine whether FGF21 was actually secreted by CMs, we analysed FGF21 protein levels in NCMs culture media. The basal rate of FGF21 secretion in media under control conditions was ›0.05 ng ml −1 24 h −1 . This basal CM FGF21 secretion rate was lower than that of mouse primary hepatocytes (›0.17 ng ml −1 24 h −1 ) [22] and brown adipocytes (›0.3 ng ml −1 24 h −1 ) [14] . After treatment with phenylephrine, the rate of FGF21 protein secretion by NCMs in culture significantly increased reaching ›0.15 ng ml −1 24 h −1 , closer to secretion rates in classical FGF21-producing cells. Next, we analysed the mechanisms controlling FGF21 expression and responsiveness in the heart in the context of hypertrophy-inducing conditions. We first studied FGF21 expression in hearts from Pparα -null mice under basal conditions and after 7 days of isoproterenol treatment ( Fig. 6e ). Cardiac FGF21 expression was reduced in Pparα -null mice under basal conditions. Isoproterenol treatment induced an increase in FGF21 mRNA expression levels in wild-type mice. However, the induction of FGF21 by isoproterenol was completely abrogated in Pparα -null mice. Co-treatment with the Sirt1 activator, resveratrol, tended to increase FGF21 expression levels in wild-type hearts, but not in Pparα -null mice. The involvement of the PPARα pathway in the control of cardiac FGF21 expression was further confirmed by treatment of NCMs with the PPARα agonist GW7647, which led to a 3.46±0.22-fold induction of FGF21 mRNA levels ( P <0.05). Next, we investigated the actions of the PPARα antagonist GW6471 on FGF21 expression in NCMs, alone and in combination with adenoviral overexpression of Sirt1 ( Fig. 6f ). Inhibition of PPARα with GW6471 significantly attenuated the increase in FGF21 transcript levels elicited by phenylephrine. Sirt1 overexpression induced an increase in FGF21 transcript levels (nearly 50-fold), an effect that was further potentiated by co-treatment with phenylephrine. Increases in FGF21 mRNA in response to Sirt1 and phenylephrine were associated with enhanced release of FGF21 protein. Such overexpression of Sirt1 in this experimental setting is known to protect against phenylephrine-induced increases in CM size and expression of ANF and α-SKA [3] . The PPARα antagonist GW6471 abolished the induction of FGF21 gene expression by phenylephrine and strongly blunted the combined effects of Sirt1 overexpression and phenylephrine treatment. Again, these effects were paralleled by changes in FGF21 protein released into the cell culture medium ( Fig. 6f ). Collectively, these results identify the Sirt1-PPARα pathway as a pivotal mechanism of control of FGF21 expression in heart. Role of endogenous production of FGF21 in cardiac cells Considering the duality of cardiac cells as both a target and a source of FGF21 and the fact that Sirt1 was the most prominent inducer of FGF21 expression, we sought to study a potential autocrine role of FGF21 by exploring the extent to which Sirt1 action on cardiac cells required the induction of FGF21 expression and release ( Fig. 7a ). Sirt1 overexpression in NCMs did not significantly modify the expression of ANF and α-SKA, as previously reported [3] , or pro-inflammatory genes ( Fig. 7a ). However, overexpression of Sirt1 significantly increased the expression levels of PGC1α, MCAD and mcpt-Iα. In order to assess the involvement of FGF21 in the actions of Sirt1, we first treated Sirt1-overexpressing NCMs with FGF21-neutralizing or control antibodies ( Supplementary Fig. S3A ). Notably, incubating NCMs with an anti-FGF21 antibody abolished the Sirt1-induced upregulation of PGC1α, MCAD and mcpt-Iα. Although Sirt1 overexpression had no effect on the expression levels of pro-inflammatory genes, the presence of FGF21-neutralizing antibody significantly increased TNFα and IL-6 mRNA levels in NCMs in the absence of Sirt1 overexpression. Moreover, blockade of FGF21 significantly induced MCP-1, TNFα and IL-6 transcript levels in the presence of overexpressed Sirt1. 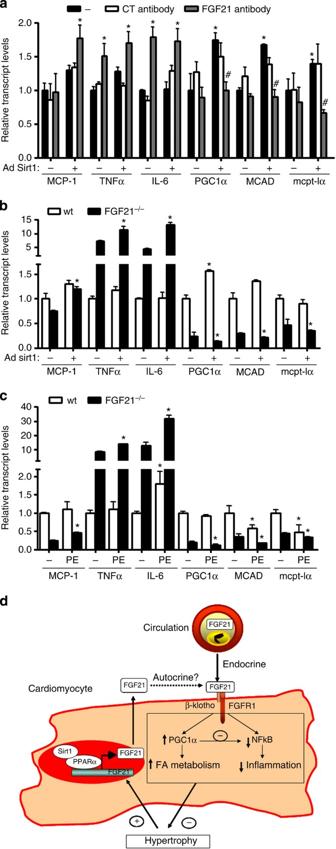Figure 7: Role of endogenous production of FGF21 in cardiac cells. (a) Rat NCMs infected with AdSirt1 or AdGFP control vector alone or with anti-FGF21 antibody or control antibody added to the culture medium. (b) Mouse NCMs from wild-type (wt, white bars) andFGF21−/−mice (black bars) infected with AdSirt1 or AdGFP control vector. (c) mRNA expression levels in mouse NCMs from wild-type andFGF21−/−mice exposed to phenylephrine (PE). Results are expressed as means±s.e.m. Each experiment was conducted in triplicate in at least two independent CM isolations. Data were analysed by one-way ANOVA (*P<0.05 compared with corresponding control cells;#P<0.05 compared with AdSirt1 infected). (d) Schematic representation of the transcriptional regulation and the actions of FGF21 in the heart. Figure 7: Role of endogenous production of FGF21 in cardiac cells. ( a ) Rat NCMs infected with AdSirt1 or AdGFP control vector alone or with anti-FGF21 antibody or control antibody added to the culture medium. ( b ) Mouse NCMs from wild-type (wt, white bars) and FGF21 −/− mice (black bars) infected with AdSirt1 or AdGFP control vector. ( c ) mRNA expression levels in mouse NCMs from wild-type and FGF21 −/− mice exposed to phenylephrine (PE). Results are expressed as means±s.e.m. Each experiment was conducted in triplicate in at least two independent CM isolations. Data were analysed by one-way ANOVA (* P <0.05 compared with corresponding control cells; # P <0.05 compared with AdSirt1 infected). ( d ) Schematic representation of the transcriptional regulation and the actions of FGF21 in the heart. Full size image In order to confirm the involvement of endogenous FGF21 expression in the actions of Sirt1 using an independent experimental approach, we next overexpressed Sirt1 in neonatal mouse CMs obtained from wild-type and Fgf21 −/− mice ( Fig. 7b and Supplementary Fig. S3B ). As in rat NCMs, Sirt1 overexpression in wild-type mouse NCMs significantly induced PGC1α, whereas it did not significantly modify the expression of pro-inflammatory marker genes. However, Sirt1 overexpression in mouse NCMs from Fgf21 −/− mice induced the expression of pro-inflammatory markers and strongly reduced PGC1α, MCAD and mcpt-Iα expression levels. Finally, we explored the role of endogenous production of FGF21 in cardiac cells by studing the effects of the hypertrophic agent phenylephrine in mouse NCMs from wild-type and Fgf21 -null mice ( Fig. 7c ). Although phenylephrine is unable to induce an increase in CM size in the mouse CM cell culture model [23] , in contrast to its actions in rat NCMs cultures, the hypertrophy-associated pro-inflammatory response is known to be mimicked in this model. In cardiac cells from wild-type mice, phenylephrine exposure significantly induced only the expression of IL-6. However, the pro-inflammatory response was dramatically enhanced in phenylephrine-treated mouse NCMs from Fgf21 −/− mice, and phenylephrine treatment of Fgf21 −/− mouse NCMs not only enhanced the induction of IL-6 but also induced a significant increase in the expression of MCP-1 and TNFα. Moreover, phenylephrine downregulated PGC1α expression only in mouse NCMs from Fgf21 −/− mice. Collectively, these data indicate that the effects of Sirt1/phenylephrine in cardiac cells require FGF21 expression and release. In the present study, we demonstrate that the heart is a target of systemic FGF21 as well as a potential source of FGF21 expression and release, as summarized in Fig. 7d . The absence of FGF21 is associated with cardiac alterations, including signs of hypertrophy, dilatation and cardiac dysfunction. A more pronounced hypertrophic response of the murine heart following isoproterenol is observed in mice lacking FGF21, whereas treatment with FGF21 protects against cardiac hypertrophy. FGF21 gene expression in cardiac cells is, in turn, stimulated by hypertrophic stimuli, and it is under the transcriptional regulation of the Sirt1-PPARα pathway. This study is the first to establish the importance of FGF21 in the heart. A few previous reports have provided some evidence that the heart is a potential target of FGF21 (refs 24 , 25 ). A recent study claimed significant cardioprotective effects of FGF21 in a mouse model of experimental MI [26] ; and a patent has been filed to exploit this therapeutic potential [27] . Our present data clearly establish that FGF21 has a strong impact on cardiac function. FGF receptors are highly expressed in the heart, as shown here and observed previously [25] . We found in heart significant levels of β-Klotho protein, the coreceptor required for the biological action of FGF21 (refs 19 , 21 ). Moreover, we found that, in cardiac cells, FGF21 induced ERK1/2 activation, the canonical mechanism known to transduce FGF21 actions on the cell surface to intracellular targets [19] , [21] . In summary, our present results are consistent with the heart being a direct target of FGF21 effects. The current findings indicate that FGF21 may exert protective effects on cardiac muscle both in vivo and in vitro . The first signs of cardiac hypertrophy developed spontaneously in Fgf21 −/− mice. The lack of other systemic alterations in the Fgf21 −/− mice strain and the very early appearance of heart alteration (propensity to hypertrophy in 6-day-old Fgf21 −/− mice) suggest that the alterations in the heart owing to FGF21 deficiency were direct. Using the continuous isoproterenol-infusion model in mice to induce cardiac hypertrophy [28] , we found that the hypertrophic response was enhanced in Fgf21 −/− mice, as evidenced by a substantially increase in the LV mass and cross-sectional area of CMs. Despite the fact that LV wall thickness was not increased in Fgf21 −/− mice compared with wild-type mice after isoproterenol treatment, we observed a marked dilatation and cardiac dysfunction in Fgf21 −/− mice, with indications of eccentric hypertrophic development. Our data also indicate that the lack of FGF21 makes the heart more prone to develop cardiac dilatation and pump dysfunction after isoproterenol treatment, features that, in wild-type mice, are known to develop only after very long-term isoproterenol administration (6 months) [28] . Results evidenced the dependence of proper cardiac function on FGF21 as an early event in the developing postnatal mouse: increased sensitization to hypertrophic induction was already present in Fgf21 −/− neonates, and normal cardiac growth could be restored by FGF21 treatment in Fgf21 −/− neonates. Notably, in newborns and adult Fgf21 −/− mice treated with isoproterenol, upregulation of pro-inflammatory markers was accompanied by a decrease in PGC1α expression levels. It has been previously shown that PGC1α is repressed by hypertrophic [29] and pro-inflammatory [30] , [31] stimuli. We show here that the inhibitory action of FGF21 on cardiac hypertrophy and inflammation was associated with the induction of PGC1α. The ability of FGF21 to induce PGC1α expression has been previously reported in adipose tissues [15] , [32] . We observed a rapid induction of CREB phosphorylation in response to FGF21, a finding in accord with previous studies on FGFR1-mediated induction of CREB in other cell types [33] . This last event may explain the fact that FGF21 induced the expression of PGC1α, a target of CREB [34] , and an established repressor of the NF-κB pro-inflammatory pathway [35] . We further report that cardiac cells are not only targets of FGF21 effects but they may also be an active site of FGF21 expression and release. Moreover, the Sirt1-PPARα pathway, which is known to be involved in the regulation of FGF21 expression in the liver in the context of the control of carbohydrate and lipid metabolism [36] , was found to have a pivotal role in controlling FGF21 expression and release in cardiac cells. Pro-inflammatory pathways are considered critical elements in the development of cardiac pathologies, such as hypertrophy and heart failure [2] . Under conditions of cardiac stress, the heart releases proteins (for example, ANF) that function in an endogenous feedback mechanism to control growth-promoting stimuli, a system that is considered to serve as a compensatory mechanism to mitigate the initial damage. Although FGF21 cardiac secretion was lower than in classical FGF21-expressing cells, FGF21 protein was substantially secreted by cardiac cells in response to cardiac stress, and cardiac FGF21 secretion was able to inhibit isoproterenol/phenylephrine-induced cardiac hypertrophic damage. The enhanced pro-inflammatory response observed in the hearts of Fgf21 −/− mice is consistent with the protective role of FGF21 under hypertrophic conditions. We obtained two lines of evidence supporting an endogenous role of FGF21 expression and secretion in cardiac cells in mediating responsiveness to Sirt1 and phenylephrine: altered responses in cardiac cells from Fgf21 −/− mice and suppression of the action of Sirt1 by FGF21 antibodies. This leads us to hypothesize that, in addition to the protective role of systemic, circulating FGF21 on the heart, the local secretion of FGF21 in the context of cardiac damage may serve as an endogenous, autoregulatory, cardioprotective signalling pathway. Confirmation of an autocrine role of cardiac FGF21 in vivo will require further experimental research based on tissue-specific FGF21 loss-of-function models. Collectively, the findings reported in this study indicate positive effects of FGF21 on the heart in the context of pathological conditions, such as the hypertrophic state. Further research is warranted to explore FGF21 as a potential tool in the development of medical strategies to prevent and/or treat cardiac damage. Animals Fgf21 −/− mice (B6N;129S5- Fgf21 tm1Lex /Mmcd) were obtained from the Mutant Mouse Regional Resource Centre (MMRRC), an NCRR-NIH-funded strain repository, and were donated to the MMRRC by Genentech, Inc. Pparα -null mice (B6.129S4- Ppara tm1Gonz /J) were obtained from Jackson laboratory (Bar Harbour, ME, USA). Wild-type littermates were used as controls for all experiments with Fgf21 -null mice and Pparα -null mice. All experiments were performed in accordance with the European Community Council directive 86/609/EEC and were approved by the Institutional Animal Care and Use Committee of the University of Barcelona. Interventions in neonatal mice Cardiac hypertrophy was induced in neonatal mice by intraperitoneally (i.p.) injecting wild-type and Fgf21 −/− mice 6-day-old neonates with isoproterenol (15 mg kg −1 per day; Sigma, St Louis, MO, USA) alone or combined with FGF21 (2.5 μg g −1 per day; Biovendor, Modrice, Czech Republic), for 7 days. Wild-type and Pparα -null mice 6-day-old neonates were injected (i.p.) with isoproterenol alone or in combination with resveratrol (RSV=50 mg kg −1 per day; Sigma), for 7 days. The effects of the inflammatory process were assessed by injecting (i.p.) 1-day-old wild-type and Fgf21 −/− neonates with LPS (5 mg Kg −1 ; Sigma) for 6 h. Isoproterenol infusion in adult mice and echocardiography Four-month-old male mice age-matched from wild-type and Fgf21 −/− mice were anesthetized with 1.5% isoflurane and subcutaneous Alzet osmotic minipumps containing PBS or isoproterenol, the latter calibrated to release the drug at a rate of 15 mg kg −1 per day for 7 days, were surgically implanted subcutaneously in the interscapular region of the mouse. This treatment did not significantly modify circulating FGF21 levels (501±42 pg ml −1 in controls versus 541±63 pg ml −1 in isoproterenol-treated mice, P =0.399). Hypertrophy was assessed by echocardiography with a Vivid Q (GE healthcare, Piscataway, NJ, USA) instrument equipped with a 12-MHz microprobe. Ventricular measurements in M-mode were made after 7 days of isoproterenol treatment. Three different cardiac cycles were measured for each assessment, and average values were obtained. Analyses of echocardiographic images were performed by two different observers in a blinded manner. Cardiac interventions in adult mice The TAC surgical procedure in mice has been performed by opening the chest and ligating the transverse aorta between the truncus brachiocephalicus and the left common carotid artery by tying a 6–0 silk suture against a 25-G (gauge) needle. Mice were killed 28 days after TAC. MI was induced by coronary artery ligation. After opening the left thorax intracostally and exposing the heart, the left descending coronary artery was ligated just proximal to its main branching point with a 6–0 polypropylene suture. Mice were killed either 5 or 28 days after MI surgery. I/R was induced by ligation of the left descending coronary artery just proximal to its main branching point with a 6–0 polypropylene suture. The suture was tied over a 3-mm long polyethylene tube (PE-10) that was left in place for 30 min. Blood flow was then re-established by removal of the tube. Mice were killed after 24 h of reperfusion. Histological analysis and detection of β-klotho Hearts were fixed for 12–24 h in 10% neutral-buffered formalin, embedded in paraffin and sectioned. Sections were deparaffinized and subsequently stained with H&E to determine CM short axis cross-sectional area in the LV. H&E-stained sections were quantified using Image J software. Fibrosis was assessed using Masson’s Trichrome staining. β-klotho expression was detected in paraffin sections by immunohistochemistry using 10 μg ml −1 of anti-β-klotho antibody (LifeSpan Biosciences, Seattle, WA, USA), according to the manufacturer’s protocol. Nuclei were stained with hematoxylin. Fatty acid oxidation Oxidation of [ 14 C]-oleic acid from freshly isolated heart homogenates was performed to assess FAO. Heart tissue was homogenized in sucrose/Tris/EDTA buffer and incubated for 60 min in reaction mixture (pH 8.0) containing [1- 14 C]-oleic acid, after which trapped CO 2 was measured. Blood pressure and heart rate Mouse blood pressure was measured using the tail-cuff method. Mice were trained on the Letica/Panlab (Barcelona, Spain) Blood Pressure Analysis System, used according to the manufacturer’s instructions for 4 days. Six consecutive measurements on the last day were averaged to calculate systolic, diastolic and mean arterial blood pressure, and heart rate. Cell culture Hearts from neonatal rats were digested with a collagenase solution (Collagenase Type I; Life Technologies Ltd, Paisley, UK) followed by differential plating to obtain the NCMs. Mouse NCMs were obtained from wild-type and Fgf21 -null mice. The experimental procedure for the culture of mouse NCMs was basically the same as that for rat NCMs. The collagenase used was type II, and instead of newborn calf serum, fetal calf serum was used. NCMs were stimulated with either the α 1 -adrenergic agonist phenylephrine (10 μmol l −1 ; Sigma), a hypertrophic growth factor, or the pro-inflammatory agent LPS (10 ng ml −1 ; Sigma). After treating for 24 h, cells were harvested for RNA isolation. Where indicated, cells were treated with the PPARα antagonist GW6471 (1 μmol l −1 ; Sigma) or FGF21 (Biovendor) for 24 h before phenylephrine exposure for additional 24 h. Antibodies against IgG (Sigma) or FGF21 (Santa Cruz Biotechnology, Inc., Santa Cruz, CA, USA) were added after the 24 h pretreatment. Isolation of adult primary CMs Excised mouse hearts were perfused with calcium-free KRB solution containing collagenase (1 mg ml −1 ) using a Langendorff perfusion apparatus until they became flaccid. The resulting cell suspension was filtered to remove undigested material, and the CM were separated from non-CMs (Non-CM) by sedimentation. Cardiac fibroblasts were isolated from neonatal wild-type mice. Briefly, excised ventricular tissues were minced into small pieces in a mixture of 0.2% collagenase type 2 and 0.25% trypsin. Minced tissue was then incubated with agitation at 37 °C for 1 h. The supernatant was collected, and the remaining tissue was immersed in digestion solution. The supernatants were pooled and filtered through a 400-μm nylon mesh filter, then centrifuged at 1,000 g for 5 min at 4 °C. The supernatant was removed, and cells were placed into fibroblast culture media and incubated for 2 h at 37 °C. Detection of myosin heavy chain in mouse NCMs by immunohistochemistry Mouse NCMs were immunostained using a specific anti-mouse myosin heavy chain antibody, developed by Fischman and colleagues (MF-20; Developmental Studies Hybridoma Bank, Iowa City, IA, USA). RNA isolation and RT–PCR Total RNA was extracted using Tripure (Roche, Indianapolis, IN, USA). RT was performed, using random hexamers primers (Applied Biosystems, Foster City, CA, USA) and 0.5 μg RNA in a total reaction volume of 20 μl. PCR was conducted in duplicate for increased accuracy. Taqman Gene Expression Assays were used ( Supplementary table S7 ), and each 25 μl of reaction mixture contained 1 μl cDNA, 12.5 μl TaqMan Universal PCR Master Mix (Applied Biosystems), 250 nM probes and 900 nM primers from Assays-on-Demand Gene Expression Assay Mix or Assays-by-Design Gene Expression Assay Mix (Applied Biosystems). Each sample was run in duplicate and the mean value was used to calculate the mRNA expression of the gene of interest and the housekeeping reference gene ( Cyclophilin A , PPIA ). The mRNA level of the gene of interest in each sample was normalized to that of the reference control using the comparative (2 −ΔCT ) method following the manufacturer’s instructions. Adenoviral-mediated gene transduction A recombinant adenovirus expressing murine Sirt1 cDNA was constructed (Ad5-CMV-Sirt1, CEBATEG, Barcelona) [37] . NCMs were infected with the Sirt1 adenoviral vector (Sirt1) or an AdCMV-GFP control vector (GFP) at 10 IFU per cell for 24 h in serum-free medium. Analysis of plasma metabolite and hormone levels Glucose and triglycerides levels were measured using the Accutrend Technology system (Roche Diagnostics, Basel, Switzerland). Free fatty acids and ketone bodies were measured using a colorimetric kit (Wako Chemicals USA Inc, Richmond, VA, USA). Leptin, insulin, IL-6, MCP-1 and resistin were quantified in 20 μl of plasma using a multiplex system (MADPK-71K, Linco Research/Millipore, Saint Charles, MO, USA) and a Luminex 100ISv2 equipment. ANF plasma levels were determined using an ELISA kit specific for ANF (Abcam, San Francisco, CA, USA). Cellular ROS levels Intracellular ROS generation was assessed using an intracellular ROS assay kit from Cell Biolabs (San Diego, CA, USA) according to the manufacture’s instructions. NF-κB activity and western blotting NF-κB activity was measured in protein extracts using the NF-κB (p65) Transcription Factor Assay kit (Cayman, Ann Arbour, MI, USA). FGF21 protein levels in NCMs culture media were detected using an FGF21 ELISA kit (Biovendor). β-Klotho protein levels were determined using specific mouse β-Klotho ELISA kits (Uscn Life Science Inc., Wuhan, China). Western blot analyses ( Supplementary table S8 ) were performed using antibodies against ERK, P-ERK, FGFR1, P-FGFR1, CREB and P-CREB (Cell Signaling Technology, Inc, Beverly, MA, USA); β-Klotho (R&D Systems, Minneapolis, MN, USA); α-tubulin (Sigma) and PGC1α (Santa Cruz). Full-length images of immunoblots are shown in Supplementary Fig. S4 . Statistics Results are presented as means±s.e.m.s. Data were analysed by one-way ANOVA, followed by Bonferroni or Dunnet’s post-hoc tests as appropriate, using GraphPad Prism (GraphPad Software Inc., San Diego, CA, USA). A P -value <0.05 was considered statistically significant. How to cite this article: Planavila, A. et al. Fibroblast growth factor 21 protects against cardiac hypertrophy in mice. Nat. Commun. 4:2019 doi: 10.1038/ncomms3019 (2013).